ALS-causative mutations in FUS/TLS confer gain and loss of function by altered association with SMN and U1-snRNP The RNA-binding protein FUS/TLS, mutation in which is causative of the fatal motor neuron disease amyotrophic lateral sclerosis (ALS), is demonstrated to directly bind to the U1-snRNP and SMN complexes. ALS-causative mutations in FUS/TLS are shown to abnormally enhance their interaction with SMN and dysregulate its function, including loss of Gems and altered levels of small nuclear RNAs. The same mutants are found to have reduced association with U1-snRNP. Correspondingly, global RNA analysis reveals a mutant-dependent loss of splicing activity, with ALS-linked mutants failing to reverse changes caused by loss of wild-type FUS/TLS. Furthermore, a common FUS/TLS mutant-associated RNA splicing signature is identified in ALS patient fibroblasts. Taken together, these studies establish potentially converging disease mechanisms in ALS and spinal muscular atrophy, with ALS-causative mutants acquiring properties representing both gain (dysregulation of SMN) and loss (reduced RNA processing mediated by U1-snRNP) of function. FUS/TLS is an hnRNP protein that contains one RNA recognition motif (RRM) and three Arginine-Glycine-Glycine-rich (RGG) motifs, the latter of which are presumably used primarily for protein–protein interactions. FUS/TLS is predominantly nuclear, but is also known to shuttle between the nucleus and cytoplasm. It has been associated with multiple steps in RNA metabolism, including transcription, splicing, microRNA processing, messenger RNA (mRNA) transport and local translation [1] . The discovery of protein aggregates and causative mutations in FUS/TLS [2] , [3] and TDP-43 (refs 4 , 5 , 6 , 7 ), two strikingly similar RBPs, as dominant causes of both the fatal adult motor neuron disease amyotrophic lateral sclerosis (ALS) and the second most frequent degenerative cognitive disorder (frontal temporal degeneration (FTD)) has initiated a paradigm shift in research on this pair of diseases, with errors in RNA maturation now a focus as a central component of disease mechanism [1] , [2] , [3] , [4] , [5] , [6] , [7] , [8] . Most disease-causing mutations are clustered in the FUS/TLS nuclear localization signal (NLS) and as expected have been shown to provoke increased cytoplasmic localization of the mutant protein [9] . However, nuclear clearance of FUS/TLS mutants does not always accompany its mutation in ALS and FTD patients [10] . More fundamentally, whether disease mechanism is driven by loss of FUS/TLS nuclear function or gain of toxicity is unsettled. Genome-wide approaches have identified thousands of RNA targets bound by FUS/TLS in vivo [11] , [12] , [13] , [14] , [15] , [16] , and depletion of it leads to broad misregulation of RNA processing, including many mRNAs encoding proteins important for neuronal function [11] . Defects in RNA metabolism also have essential roles in the childhood-onset motor neuron disease spinal muscular atrophy (SMA) caused by deficiency of the SMN protein [17] . SMN is part of a large multiprotein complex that is essential for the biogenesis of small nuclear ribonucleoprotein particles (snRNPs) [18] , [19] , [20] . As core components of the spliceosome, snRNPs are comprised of small nuclear RNAs (snRNAs) (U1, U2, U4, U5 and U6 for the major spliceosome; U11, U12, U4atac, U5, and U6atac for the minor spliceosome) and their bound proteins. snRNPs function to define splice sites and catalyse RNA splicing reactions [21] . Prior efforts have reported markedly decreased snRNP assembly activity and reduced snRNA levels in SMN-deficient cells [22] , [23] , [24] , [25] , SMA mice [24] , [25] , [26] , [27] and SMA patient tissues [22] , [27] , thereby producing broadly misregulated RNA splicing [24] , [25] . SMN complexes are primarily localized in the cytoplasm, in intranuclear Gems, and in axons of motor neurons [28] . Loss of Gems is a cellular hallmark in SMA. Both reduction and mutation in TDP-43 or SOD1 have been reported in mice to disrupt Gem assembly or stabilization [29] , [30] , [31] , [32] . FUS/TLS, too, has been reported to be associated with SMN complexes [33] , [34] , [35] . Gems and axonal distribution of SMN are reduced (about 50 and 20%, respectively) in patient fibroblasts or transfected rat cortical neurons with ALS-associated mutations in FUS/TLS [33] , [35] . Cytosolic mislocalization of FUS/TLS mutants has also been shown to increase snRNA accumulation within the cytoplasm [36] . However, the molecular mechanism(s) underlying such changes is not well established. Here we determine that FUS/TLS directly binds the SMN protein, with its association mediated by the RGG motifs in FUS/TLS and the Tudor domain in SMN. Surprisingly, multiple ALS-causative mutations in FUS/TLS increase FUS/TLS interaction with SMN, thereby affecting the normal function of SMN by both reducing Gem bodies and changing steady-state levels of some snRNAs in transgenic mouse tissues and patient fibroblasts expressing mutant FUS/TLS. Furthermore, FUS/TLS is found to interact with U1-snRNP complexes, with ALS-causative mutations shown to reduce this binding. Global analysis of RNA splicing reveals that mutant FUS/TLS-dependent splicing changes mimic partial FUS/TLS loss of activity, independent of cytosolic mislocalization. A common RNA splicing signature is identified in patient fibroblasts carrying different FUS/TLS mutations, with many changes overlapping ones induced by reducing either FUS/TLS or SMN. These results provide evidence for both gain and loss of function caused by ALS-linked mutations in FUS/TLS and the potential convergence in pathological pathways of ALS and SMA. Identification of a FUS/TLS protein interaction network We sought to comprehensively determine FUS/TLS-associated proteins by combining tandem affinity purification (TAP) with quantitative mass spectrometric analysis using stable isotope labelling by amino acids in cell culture (SILAC) [37] ( Fig. 1 ). FUS/TLS was triply tagged, including a localization affinity purification (LAP)-tag (comprised of green fluorescent protein (GFP) and hexa-histidine tags for visualization and purification) and an additional amino-terminal haemagglutinin (HA) (YPYDVPDYA) tag ( Fig. 1a ). A HeLa cell line stably expressing a single copy of LAP-tagged FUS/TLS was generated using a site-directed recombinase (Flip). Epitope-tagged human FUS/TLS accumulated to a level equivalent to endogenous FUS/TLS in the parental cells, with a corresponding reduction in untagged endogenous FUS/TLS to about half its initial level, presumably through autoregulation ( Fig. 1b ) [11] , [38] . Tagged wild-type FUS/TLS accumulated within nuclei in a pattern indistinguishable from endogenous FUS/TLS ( Fig. 1c ). 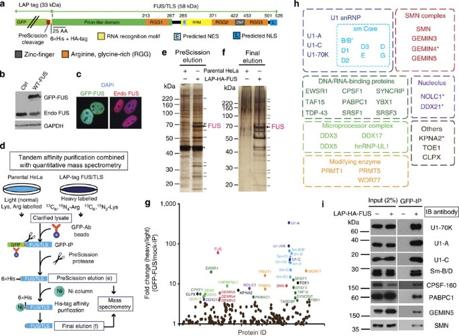Figure 1: Quantitative proteomic analysis of FUS/TLS using stable isotope labelling by amino acids in cell culture (SILAC) coupled with tandem affinity purification (TAP). (a) Schematic representation of FST/TLS tagging including the localization and affinity purification (LAP)-tag composed of GFP followed by PreScission protease cleavage sequences, a 6 × histidine-tag, and an HA-peptide (YPYDVPDYA). (b) Immunoblotting of FUS/TLS showed comparable levels of cell extracts for GFP-tagged or endogenous FUS/TLS. (c) GFP fluorescence of induced GFP-tagged FUS/TLS and immunofluorescence of endogenous FUS/TLS on HeLa Flp-In cells. (d) Schematic representation of TAP purification and quantitative analysis using SILAC. (e,f) Silver stain of the samples from the PreScission (e) and final (f) elutions of the tandem affinity purification steps. Arrow indicates tagged FUS/TLS and * denoted GST-tagged PreScission protease; positions of other visible polypeptides are marked with dashes. (g) Graphic representation of FUS/TLS interactome.Yaxis displays the average ratio of different peptides per identified protein; thexaxis displays the protein ID in alphabetical order, with a fourfold enrichment above background signal considered to be a FUS/TLS-associated protein (highlighted in colours that match identities inh). (h) Summary of FUS/TLS-associated proteins, identified with peptides containing only heavy Lys/Arg and by multiple different peptides from at least two independent runs, except *, which denotes the proteins were identified only in one run. The associated proteins were grouped according to the known assigned functions for each. (i) Confirmation of putative FUS/TLS-associating proteins by immunoblotting, including U1-70K, U1-A, U1-C, Sm-B/D, CPSF-160, PABPC1, GEMIN5 and SMN. DAPI, 4,6-diamidino-2-phenylindole. Figure 1: Quantitative proteomic analysis of FUS/TLS using stable isotope labelling by amino acids in cell culture (SILAC) coupled with tandem affinity purification (TAP). ( a ) Schematic representation of FST/TLS tagging including the localization and affinity purification (LAP)-tag composed of GFP followed by PreScission protease cleavage sequences, a 6 × histidine-tag, and an HA-peptide (YPYDVPDYA). ( b ) Immunoblotting of FUS/TLS showed comparable levels of cell extracts for GFP-tagged or endogenous FUS/TLS. ( c ) GFP fluorescence of induced GFP-tagged FUS/TLS and immunofluorescence of endogenous FUS/TLS on HeLa Flp-In cells. ( d ) Schematic representation of TAP purification and quantitative analysis using SILAC. ( e , f ) Silver stain of the samples from the PreScission ( e ) and final ( f ) elutions of the tandem affinity purification steps. Arrow indicates tagged FUS/TLS and * denoted GST-tagged PreScission protease; positions of other visible polypeptides are marked with dashes. ( g ) Graphic representation of FUS/TLS interactome. Y axis displays the average ratio of different peptides per identified protein; the x axis displays the protein ID in alphabetical order, with a fourfold enrichment above background signal considered to be a FUS/TLS-associated protein (highlighted in colours that match identities in h ). ( h ) Summary of FUS/TLS-associated proteins, identified with peptides containing only heavy Lys/Arg and by multiple different peptides from at least two independent runs, except *, which denotes the proteins were identified only in one run. The associated proteins were grouped according to the known assigned functions for each. ( i ) Confirmation of putative FUS/TLS-associating proteins by immunoblotting, including U1-70K, U1-A, U1-C, Sm-B/D, CPSF-160, PABPC1, GEMIN5 and SMN. DAPI, 4,6-diamidino-2-phenylindole. Full size image To identify specific interactors, even those in low abundance while eliminating abundant contaminant proteins, cell lines stably expressing the LAP-tag-containing wild-type FUS/TLS were grown in isotopically ‘heavy’ medium containing 13 C 6 , 15 N 4 -arginine and 13 C 6 , 15 N 2 -lysine, while the parental line (that is, no transgene) was grown in ‘light’ medium containing normal arginine and lysine ( Fig. 1d ). Compared with the parental cells, the first prescission cleavage eluates after GFP immunoprecipitation, and final eluates after His-tag affinity chromatography of extracts from cells expressing the tagged wild-type human FUS/TLS contained at least 11 and 17, respectively, additional polypeptides that were observable directly with silver staining (marked with dashed lines, Fig. 1e,f ). Quantitative mass spectrometry was used to identify these FUS/TLS-associated proteins. The criteria for protein identification included (1) a calculated false discovery rate [39] below 1%, (2) all the proteins must have been identified with more than two unique peptides and (3) all peptide signals (heavy/light isotope labelling) for each protein must have at least a fourfold enrichment in FUS/TLS immunoprecipitates compared with the LAP control (purified from the parental HeLa cell line). With these criteria, the FUS/TLS interactome was found to be comprised of 35 proteins ( Fig. 1g,h ). All of these are proteins involved in RNA processing: (a) associated components of the U1-snRNP and SMN complexes, (b) known splicing factors (SFSR1 and SFSR3), (c) other ALS-linked RBPs (EWSR1, TAF-15 and TDP-43), (d) associated with polyadenylation (CPSF-160 (cleavage and polyadenylation-specific factor 1, 160 kDa) and PABPC1 (cytoplasmic poly(A)-binding protein 1)) and (e) components of the Drosha microprocessing complex (DDX3, DDX5, DDX17 and hnRNP-U1-like protein) essential for microRNA biogenesis. Using immunoblotting, components of U1-snRNP (U1-70K, U1-A, U1-C and sm-B/D), SMN (Gemin 5 and SMN) and polyadenylation (CPSF-160 and PABP) were confirmed to be selectively present in the FUS/TLS affinity purified fraction of the LAP-tagged FUS/TLS-expressing cell extracts ( Fig. 1i ). The complete list of FUS/TLS immunoprecipitated proteins is presented in Supplementary Table 1 . FUS/TLS interacts with SMN in cells and mouse tissues To further test the association between FUS/TLS and SMN, endogenous FUS/TLS was immunoprecipitated from extracts of HeLa cells and mouse neuroblastoma (N2a) cells either undifferentiated or 5 days after differentiation into a neuron-like morphology. In each case, a proportion of SMN co-precipitated with FUS/TLS, with an enhanced interaction in the neuron-like cells independent of differentiation status ( Fig. 2a ). Similarly, FUS/TLS was found complexed with SMN in multiple mouse tissues, with comparable co-precipitation with SMN in liver, brain and spinal cord extracts ( Supplementary Fig. 1a ). The immunoprecipitation was specific to FUS/TLS interacting proteins, as an unrelated protein, glyceraldehyde 3-phosphate dehydrogenase (GAPDH), was not co-purified ( Supplementary Fig. 1b ). 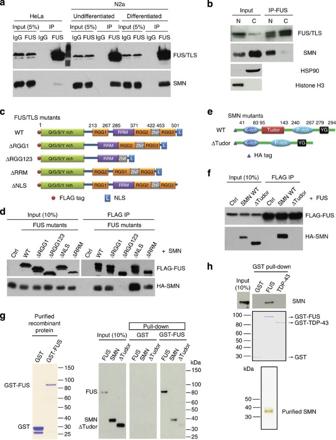Figure 2: FUS/TLS interacts with SMN through Arginine-Glycine-Glycine-rich (RGG) motifs and the Tudor domain. (a) Immunoprecipitation was carried out from whole-cell lysates of HeLa, undifferentiated and differentiated N2a cells using Protein G Dynabeads coated with control immunoglobulin (IgG) or FUS/TLS polyclonal antibody. The input and precipitated proteins were immunoblotted with FUS/TLS and SMN monoclonal antibodies. (b) N2a cells were fractionated to separate nucleus and cytoplasm. FUS/TLS was immunoprecipitated from each fraction, followed by immunoblotting with SMN antibody. HSP90 and histone H3 were used as cytosol and nuclear markers, respectively. (c) Diagrams of the FLAG-tagged FUS/TLS deletion mutants. (d) HeLa cells were co-transfected with various FLAG-tagged FUS/TLS cDNAs and the HA-tagged SMN construct. Immunoprecipitation was carried out using anti-FLAG M2 beads followed by immunoblotting with FLAG and HA antibodies. (e) Diagrams of the HA-tagged SMN constructs. (f) HeLa cells were co-transfected with FLAG-tagged FUS/TLS cDNA and HA-tagged SMN mutants. Immunoprecipitation/immunoblotting was performed as ind. (g) GST and GST-FUS were expressed and purified from bacteria, separated on SDS–PAGE and stained with Coomassie blue (left). Purifed GST or GST-FUS was incubated with35S-labelled FUS/TLS, SMN and SMN ΔTudor synthesized byin vitrotranscription and translation, together with glutathione sepharose. The associated proteins were analysed by autoradiography. (h) Purified GST, GST-FUS and GST-TDP-43 were separated on SDS–PAGE and stained with Coomassie blue (middle). The three proteins were incubated with purified recombinant SMN (bottom)in vitroand GST complexes were affinity purified with glutathionine beads, seperated on SDS–PAGE and immunoblotted with SMN antibody (top). Figure 2: FUS/TLS interacts with SMN through Arginine-Glycine-Glycine-rich (RGG) motifs and the Tudor domain. ( a ) Immunoprecipitation was carried out from whole-cell lysates of HeLa, undifferentiated and differentiated N2a cells using Protein G Dynabeads coated with control immunoglobulin (IgG) or FUS/TLS polyclonal antibody. The input and precipitated proteins were immunoblotted with FUS/TLS and SMN monoclonal antibodies. ( b ) N2a cells were fractionated to separate nucleus and cytoplasm. FUS/TLS was immunoprecipitated from each fraction, followed by immunoblotting with SMN antibody. HSP90 and histone H3 were used as cytosol and nuclear markers, respectively. ( c ) Diagrams of the FLAG-tagged FUS/TLS deletion mutants. ( d ) HeLa cells were co-transfected with various FLAG-tagged FUS/TLS cDNAs and the HA-tagged SMN construct. Immunoprecipitation was carried out using anti-FLAG M2 beads followed by immunoblotting with FLAG and HA antibodies. ( e ) Diagrams of the HA-tagged SMN constructs. ( f ) HeLa cells were co-transfected with FLAG-tagged FUS/TLS cDNA and HA-tagged SMN mutants. Immunoprecipitation/immunoblotting was performed as in d . ( g ) GST and GST-FUS were expressed and purified from bacteria, separated on SDS–PAGE and stained with Coomassie blue (left). Purifed GST or GST-FUS was incubated with 35 S-labelled FUS/TLS, SMN and SMN ΔTudor synthesized by in vitro transcription and translation, together with glutathione sepharose. The associated proteins were analysed by autoradiography. ( h ) Purified GST, GST-FUS and GST-TDP-43 were separated on SDS–PAGE and stained with Coomassie blue (middle). The three proteins were incubated with purified recombinant SMN (bottom) in vitro and GST complexes were affinity purified with glutathionine beads, seperated on SDS–PAGE and immunoblotted with SMN antibody (top). Full size image Wild-type FUS/TLS is predominantly nuclear, as demonstrated by immunoblotting of equal proportions of nuclear and cytoplasmic fractions ( Fig. 2b ), but is thought to shuttle between the nucleus and cytoplasm [40] . In both fibroblasts and neuroblastoma cells, endogenous SMN was primarily cytoplasmic, diffusely found throughout the cytoplasm in addition to accumulation in bright intranuclear foci (Gems) ( Supplementary Fig. 1c ). Immunoprecipitation from nuclear and cytoplasmic extracts from N2a cells revealed that wild-type FUS/TLS associated almost exclusively with nuclear, not cytoplasmic, SMN ( Fig. 2b ). The RGG and Tudor domains are essential for the interaction Methylated arginines in RGG motifs are recognized by Tudor domains, a ~60-amino-acid structure proposed to facilitate protein–protein interactions involved in several RNA processing pathways [41] . Since SMN contains a single Tudor domain and interacts with several RG-containing proteins, including Ewing’s sarcoma protein (EWS) (a homologue of FUS/TLS [42] ), we tested whether the RGG motifs of FUS/TLS mediate the association with SMN. Deletion mutants of FUS/TLS ( Fig. 2c ) and SMN ( Fig. 2e ) were generated to identify which domain(s) mediates their interaction. FLAG-tagged FUS/TLS and HA-tagged SMN were expressed in HeLa cells using DNA transfection, extracts were prepared, FUS/TLS-containing complexes were recovered with FLAG antibody and finally any co-purified SMN was detected with an HA antibody. While deletion of a single RGG motif from FUS/TLS was insufficient to eliminate co-precipitation of SMN, deletion of all three RGG motifs (producing ΔRGG123) abolished complex assembly containing both FUS/TLS and SMN ( Fig. 2d ). However, because the decreased association of the ΔRGG123 mutant with SMN also correlated with its mislocalization in the cytoplasm ( Supplementary Fig. 1d ) and the normal interaction is found predominantly intranuclearly ( Fig. 2b ), we then deleted the NLS sequences (at the FUS/TLS C terminus) but kept the RGG motifs intact ( Fig. 2c ) so as to test whether loss of interaction was influenced by cytosolic mislocalization of FUS/TLS. ΔNLS and ΔRGG123 mutants distributed cytoplasmically in similar patterns ( Supplementary Fig. 1d ). The ΔNLS mutant associated with a substantially higher proportion of SMN than did wild-type FUS/TLS ( Fig. 2d ), implicating an increased cytoplasmic concentration driving an enhanced, cytosolic interaction with SMN. FUS/TLS remained complexed to SMN even when its RRM was deleted ( Fig. 2d ). The Tudor domain of SMN was essential for this interaction, as SMN was no longer co-immunoprecipitated with FUS/TLS when the Tudor domain was deleted ( Fig. 2f ). Incubation of purified recombinant glutatione S-transferase (GST)-tagged FUS/TLS protein with 35 S-labelled FUS/TLS or SMN protein synthesized by coupled in vitro transcription and translation demonstrated that GST-FUS bound to itself or to wild-type SMN. GST alone bound neither, as expected. The Tudor domain in SMN was required for binding to FUS/TLS ( Fig. 2g ). Incubation of purified His-tagged recombinant SMN with purified recombinant GST, GST-tagged FUS/TLS or GST-tagged TDP-43 revealed that GST-FUS, but not GST or GST-TDP-43, bound SMN directly ( Fig. 2h ). RNase treatment of N2a cell lysates eliminated co-immunoprecipitation ( Supplementary Fig. 1e ), supporting an RNA-mediated enhancement of FUS/TLS interaction with SMN. Mutants in FUS alter interaction with SMN and reduce Gems FUS/TLS-causative mutations in ALS cluster in two locations. Most lie in the NLS sequence at the C terminus, with most of the others within the RGG motifs [8] . Deletions within either region affect the association with SMN ( Fig. 2 ). To test how ALS-linked mutations in FUS/TLS affected its association with SMN, we co-transfected HeLa cells with genes encoding FLAG-tagged, wild-type or mutant FUS/TLS and HA-tagged SMN. FUS/TLS immunoprecipitates revealed that five of six mutations in the NLS (except R521H) increased binding to SMN ( Fig. 3a , lanes 5–10), while mutants within the RGG motifs had the opposite effect ( Fig. 3a , lanes 3 and 4). The most marked increase in SMN binding was induced by the truncation mutant R495X, which lacks the complete NLS sequence. 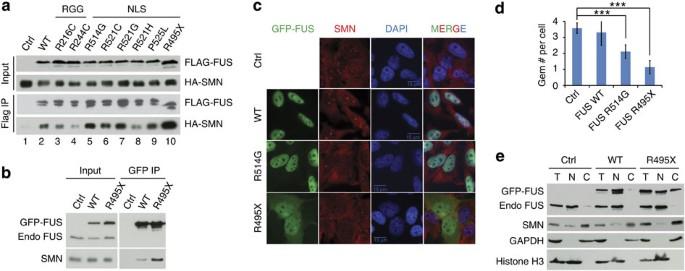Figure 3: ALS-causative mutations of FUS/TLS alter interaction with SMN and reduce Gem number. (a) HeLa cells were co-transfected with FLAG-tagged FUS/TLS carrying ALS-linked mutations and HA-tagged SMN cDNA, extracts prepared and FUS/TLS immunoprecipitated with FLAG antibody, followed by immunoblotting with HA antibody. (b) GFP immunoprecipitation from HeLa Flp-In cells expressing GFP-tagged wild-type or R495X mutant FUS/TLS, followed by immunoblotting with FUS/TLS (Santa Cruz) or SMN antibody. (c) GFP fluorescence and SMN immunofluorescence of HeLa Flp-In cells induced to express GFP-tagged wild-type or ALS-linked mutant FUS/TLS. Gems were detected with SMN antibody (red spots in nucleus). (d) Quantification of Gem numbers per cell inc. More than 100 cells were counted in each condition. (***P<0.001, one-way analysis of variance using thepost hoctest; error bars represent s.d.) (e) HeLa Flp-In cells were induced with tetracycline to express GFP-tagged wild-type or R495X FUS/TLS transgenes. Cells were fractionated to separate nucleus and cytoplasm. Equal proportion of cell extracts from total, nuclear and cytosol fractions were immunoblotted with FUS/TLS, SMN, GAPDH (cytosol marker) and histone H3 (nuclear marker) antibodies. WT, wild type. Figure 3: ALS-causative mutations of FUS/TLS alter interaction with SMN and reduce Gem number. ( a ) HeLa cells were co-transfected with FLAG-tagged FUS/TLS carrying ALS-linked mutations and HA-tagged SMN cDNA, extracts prepared and FUS/TLS immunoprecipitated with FLAG antibody, followed by immunoblotting with HA antibody. ( b ) GFP immunoprecipitation from HeLa Flp-In cells expressing GFP-tagged wild-type or R495X mutant FUS/TLS, followed by immunoblotting with FUS/TLS (Santa Cruz) or SMN antibody. ( c ) GFP fluorescence and SMN immunofluorescence of HeLa Flp-In cells induced to express GFP-tagged wild-type or ALS-linked mutant FUS/TLS. Gems were detected with SMN antibody (red spots in nucleus). ( d ) Quantification of Gem numbers per cell in c . More than 100 cells were counted in each condition. (*** P <0.001, one-way analysis of variance using the post hoc test; error bars represent s.d.) ( e ) HeLa Flp-In cells were induced with tetracycline to express GFP-tagged wild-type or R495X FUS/TLS transgenes. Cells were fractionated to separate nucleus and cytoplasm. Equal proportion of cell extracts from total, nuclear and cytosol fractions were immunoblotted with FUS/TLS, SMN, GAPDH (cytosol marker) and histone H3 (nuclear marker) antibodies. WT, wild type. Full size image We then used HeLa cell lines with an integrated single copy, tetracycline-inducible wild-type or mutant-GFP-tagged FUS/TLS gene. Induction produced levels 2–3 times of endogenous FUS/TLS ( Fig. 3b ). The truncation mutant R495X was mislocalized, with a clearly identifiable presence in the cytoplasm ( Fig. 3c ; Supplementary Fig. 2 ). Relative to wild-type FUS/TLS, mutation in the NLS (R495X) produced an approximately threefold increased binding between exogenously expressed FUS/TLS and endogenous SMN (using GFP immunoprecipitation) ( Fig. 3b ), confirming at nearly physiological levels of accumulation what was previously seen with higher levels ( Fig. 3a ). Analysis of immunostaining with an SMN antibody revealed that in cells expressing a wild-type FUS/TLS transgene, the number of nuclear Gems was unchanged relative to cells without a transgene. However, accompanying its cytosolic mislocalization, expression of ALS-linked R495X mutant strikingly reduced nuclear Gems ( Fig. 3c ; quantified in Fig. 3d ). To test the possibility that the loss of nuclear Gems was mediated by mutant FUS/TLS sequestering SMN in the cytoplasm, FUS/TLS variant R495X was induced and the cells fractionated into nuclear and cytoplasmic components. Cytosolic GAPDH and nuclear histone H3 confirmed the fractionation purity ( Fig. 3e ). Both endogenous and transgenic wild-type FUS/TLS were mainly nuclear, but approximately one-third of the R495X mutant was cytoplasmic ( Fig. 3e ). An increased proportion of SMN was relocalized to the cytoplasm in the presence of FUS/TLS R495X ( Fig. 3e ), consistent with mislocalization of FUS/TLS altering the distribution of SMN and thereby affecting Gem assembly/stability in the nucleus. Note, however, that while Gem reduction was a common property of all tested ALS-linked FUS/TLS mutants, cytoplasmic redistribution of FUS/TLS was not essential, as it was also seen upon accumulation of the almost exclusively nuclear R514G ( Fig. 3c,d ; Supplementary Fig. 2 ). It is possible the abnormal interaction of mutant FUS/TLS with SMN affects overall SMN dynamics within nuclei. Reduction of Gems and altered snRNAs in patient fibroblasts We next examined Gem formation in ALS patient fibroblast lines carrying FUS/TLS mutations. In lines with R521G or H517Q mutations, Gem numbers per cell were modestly reduced relative to control cell lines from three different individuals ( Fig. 4a,b ), albeit there was no obvious increase in cytoplasmic accumulation of FUS/TLS ( Supplementary Fig. 3 ). In contrast, the frameshift mutation (M511Nfs*6) that leads to deletion of the NLS was diffusely localized in both the cytoplasm and nucleus, and Gem bodies were markedly reduced ( Fig. 4a,b ), consistent with our findings in HeLa cells that the FUS/TLS NLS truncation mutant had the most severe phenotype ( Fig. 3 , comparable to the R495X mutation). 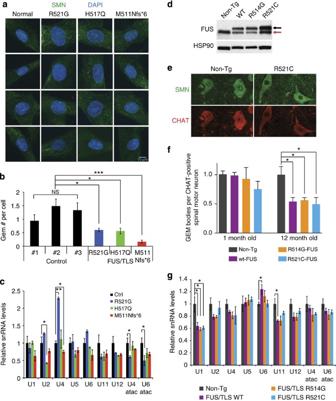Figure 4: Reduction of Gems and changes in snRNA levels in ALS patient fibroblasts and transgenic mouse spinal cords. (a) Representative images of Gem bodies stained with SMN antibody in human fibroblasts from normal or ALS patient carrying FUS/TLS mutations. (b) Quantification of average Gem numbers per cell ina, from three independent experiments. (NSP=0.084 for variance among the three control fibroblasts by one-way analysis of variance (ANOVA); *P<0.01 and ***P<0.0005 for mutants versus controls, one-way ANOVA using thepost hoctest; error bars represent s.d.) (c) qRT–PCR of U-snRNAs in normal and patient fibroblast harbouring FUS/TLS mutations. The control is the average of three normal fibroblast cell lines. Each condition has three biological replicates. The group variance for each gene was analysed by one-way ANOVA. The genes with significant variences (P<0.05) were further analysed using thepost hoctest comparing mutants versus control (*P<0.05, **P<0.001, error bars represent s.e.m.) (d) Immunoblotting of whole-spinal cord lysates from transgenic mice with mouse/human FUS/TLS antibody. (e) Representative images of Gem bodies in the motor neurons at the lumbar section of the spinal cord in mice at the symptomatic (12 month) stage. Nuclear Gem bodies were visualized using SMN antibody and motor neurons were stained with ChAT (choline acetyl-transferase) antibody. Left and right panels show representative images from non-transgenic littermate controls and R521C-FUS expressing transgenic mice. (f) Quantification of average Gem numbers per motor neuron in control or transgenic mice expressing human wild-type, R514G or R521C mutations at 1 month and 12 months of age with three biological replicates in each group (*P<0.05, one-way ANOVA using thepost hoctest; error bars represent s.e.m.) (g) qRT–PCR of U-snRNAs in spinal cord of mice at 12 months carrying no transgene, or FUS/TLS wild-type, R514G, R521C mutant transgenes. Each condition has three biological replicates (*P<0.05, one-way ANOVA using thepost hoctest; error bars represent s.e.m.). NS, not significant. Figure 4: Reduction of Gems and changes in snRNA levels in ALS patient fibroblasts and transgenic mouse spinal cords. ( a ) Representative images of Gem bodies stained with SMN antibody in human fibroblasts from normal or ALS patient carrying FUS/TLS mutations. ( b ) Quantification of average Gem numbers per cell in a , from three independent experiments. (NSP=0.084 for variance among the three control fibroblasts by one-way analysis of variance (ANOVA); * P <0.01 and *** P <0.0005 for mutants versus controls, one-way ANOVA using the post hoc test; error bars represent s.d.) ( c ) qRT–PCR of U-snRNAs in normal and patient fibroblast harbouring FUS/TLS mutations. The control is the average of three normal fibroblast cell lines. Each condition has three biological replicates. The group variance for each gene was analysed by one-way ANOVA. The genes with significant variences ( P <0.05) were further analysed using the post hoc test comparing mutants versus control (* P <0.05, ** P <0.001, error bars represent s.e.m.) ( d ) Immunoblotting of whole-spinal cord lysates from transgenic mice with mouse/human FUS/TLS antibody. ( e ) Representative images of Gem bodies in the motor neurons at the lumbar section of the spinal cord in mice at the symptomatic (12 month) stage. Nuclear Gem bodies were visualized using SMN antibody and motor neurons were stained with ChAT (choline acetyl-transferase) antibody. Left and right panels show representative images from non-transgenic littermate controls and R521C-FUS expressing transgenic mice. ( f ) Quantification of average Gem numbers per motor neuron in control or transgenic mice expressing human wild-type, R514G or R521C mutations at 1 month and 12 months of age with three biological replicates in each group (* P <0.05, one-way ANOVA using the post hoc test; error bars represent s.e.m.) ( g ) qRT–PCR of U-snRNAs in spinal cord of mice at 12 months carrying no transgene, or FUS/TLS wild-type, R514G, R521C mutant transgenes. Each condition has three biological replicates (* P <0.05, one-way ANOVA using the post hoc test; error bars represent s.e.m.). NS, not significant. Full size image The SMN complex has been well established to act in the cytoplasm as a chaperone-catalysing assembly of snRNPs, essential components of the spliceosome [18] . SMN deficiency is known to severely decrease snRNP assembly capacity and cause profound alterations in snRNA levels [24] , [27] , although the extent of changes in different snRNAs varies in different cell types and tissues of SMA patients [24] , [27] . The nuclear function of Gems is not clear, beyond some evidence for partial (and dynamic) association with Cajal bodies [43] , [44] , [45] , a nuclear structure involved in snRNP maturation and recycling [46] . To test whether ALS-causing FUS/TLS mutants affected snRNP metabolism, we compared the snRNA levels in ALS patient fibroblasts harbouring FUS/TLS mutations with levels in normal control fibroblasts. Although variations were found among the lines with different mutations, quantitative reverse transcription (qRT)–PCR measurement revealed a trend for reduced snRNAs of both major and minor classes in the patient-derived cells with the exception of R521G, which increased several snRNAs of the major class, particularly U4, accompanied by reduced snRNAs in the minor class ( Fig. 4c ). Reduction of Gems and altered snRNAs in FUS transgenic mice To further determine whether a decrease in Gem bodies is a common and relevant feature in FUS/TLS-mediated toxicity in vivo , we examined two different sets of FUS/TLS transgenic mouse models that develop age-dependent loss of lower motor neurons. The first set of FUS/TLS mice express HA-tagged complementay DNAs (cDNAs) encoding wild type or either of the two ALS-linked mutations (R514G and R521C) in human FUS/TLS that are transcribed from a mouse prion promoter (to be reported in detail elsewhere). Co-labelling for the motor neuron marker choline acetyl-transferase and for SMN revealed that at 1 month of age, an age prior to development of pathology or abnormal motor phenotypes, expression of mutant R521C had already provoked a slight reduction of Gems ( Fig. 4d–f ). By 12 months of age, all transgenic lines had developed abnormal motor symptoms with about 25% denervation and α-motor neuron loss, and this was accompanied by 40–50% reduction in Gems in motor neurons ( Fig. 4f ; P =0.03, 0.05 and 0.04 for R521C, R514G and wild-type, respectively). Thus, in all of these transgenic mouse lines there is age-dependent loss of Gems that correlates with appearance of symptoms ( Fig. 4f ). Analysis of an additional FUS/TLS transgenic mouse line (in which a hamster prion promoter was used to drive expression of a FLAG-tagged human FUS cDNA with the R521C mutation [47] ) revealed a marked reduction (20-fold; P =0.0001) in GEM numbers at a symptomatic stage ( Supplementary Fig. 4 ). Furthermore, analysis of snRNA levels revealed that U1 and U11 snRNAs were the most reduced (by 40 and 20%, respectively) in the mutant transgenic mice compared with non-transgenic littermates ( Fig. 4g ). Mutations of FUS/TLS reduce interaction with U1-snRNP Association of FUS/TLS with U1-snRNP identified earlier by mass spectrometry ( Fig. 1g–i ) was further confirmed by reciprocal immunoprecipitation: GFP-tagged FUS/TLS pulled down FLAG-tagged U1-70K and U1-A, and FLAG-tagged U1-70K and U1-A pulled down both GFP-tagged and endogenous FUS/TLS ( Fig. 5a,b ). Similarly, U1-70K and U1-A co-immunoprecipitated with CPSF-160, a protein involved in 3′-end processing of mRNAs ( Fig. 5b ). U1-C failed to do so in this assay, possibly because the FLAG tag on this small (17 kD) protein affected its proper incorporation into the U1-snRNP complex and interaction with FUS/TLS. The interaction was RNA dependent, as RNase treatment eliminated co-immunoprecipitation ( Supplementary Fig. 5 ). Furthermore, FUS/TLS, SMN, CPSF-160 and components of U1-snRNP, including U1-70K and U1-A, precisely eluted in the same (~1.8 MkDa) gel permeation chromatography fractions ( Fig. 5c ). In contrast, PRMT1 (protein arginine methyl-transferase 1), another FUS/TLS interactor, migrated together with FUS/TLS at fractions corresponding to between 670 and 440 kDa, fractions that did not contain U1 components ( Fig. 5c ). 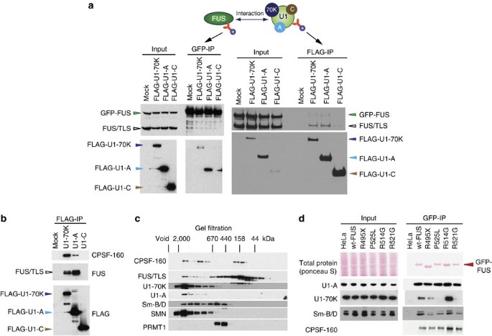Figure 5: ALS-linked mutations in FUS/TLS reduce its interaction with U1-snRNP. (a) Association of FUS/TLS with specific factors of U1-snRNP. FLp-In cells expressing wild-type FUS/TLS were transiently transfected with FLAG-tagged U1-70K, U1-A or U1-C and immunoprecipiations performed for FUS/TLS or U1-70K, U1-A or U1-C using antibodies to the Lap or FLAG tags, and finally assayed by immunoblotting for FUS or FLAG-tagged U1 components. (b) Association of FUS/TLS with U1-snRNP and CPSF-160 was assayed by immunoprecipitation with FLAG antibodies of extracts from FLAG-tag U1-70K- or U1-A-expressing cells, and then immunoblotted for endogenous FUS/TLS and CPSF-160. (c) Size-exclusion chromatography of extracts of cells transfected as ina. Estimated molecular weights are indicated at the top using blue detran (2 MDa), thyroglobulin (670 kDa), ferritin (440 kDa), aldolase (158 kDa) and ovalbumin (44 kDa) as markers. Collected fractions were analysed on SDS–PAGE and immunoblotted with CPSF-160, FUS/TLS, U1-70K, U1-A, Sm-B/D, SMN and PRMT1 antibodies. (d) Reduced association between U1-snRNP with ALS-linked mutations in FUS/TLS. Extracts of isogenic lines expressing different GFP-tagged ALS-linked FUS/TLS mutations were immunoprecipiated with GFP antibodies and immunoblotted with antibodies against U1-A, U1-70K, Sm-B/D or CPSF-160. Decreased association of U1-70K and Sm-B/D with FUS/TLS was apparent in three of the four NLS mutations. Figure 5: ALS-linked mutations in FUS/TLS reduce its interaction with U1-snRNP. ( a ) Association of FUS/TLS with specific factors of U1-snRNP. FLp-In cells expressing wild-type FUS/TLS were transiently transfected with FLAG-tagged U1-70K, U1-A or U1-C and immunoprecipiations performed for FUS/TLS or U1-70K, U1-A or U1-C using antibodies to the Lap or FLAG tags, and finally assayed by immunoblotting for FUS or FLAG-tagged U1 components. ( b ) Association of FUS/TLS with U1-snRNP and CPSF-160 was assayed by immunoprecipitation with FLAG antibodies of extracts from FLAG-tag U1-70K- or U1-A-expressing cells, and then immunoblotted for endogenous FUS/TLS and CPSF-160. ( c ) Size-exclusion chromatography of extracts of cells transfected as in a . Estimated molecular weights are indicated at the top using blue detran (2 MDa), thyroglobulin (670 kDa), ferritin (440 kDa), aldolase (158 kDa) and ovalbumin (44 kDa) as markers. Collected fractions were analysed on SDS–PAGE and immunoblotted with CPSF-160, FUS/TLS, U1-70K, U1-A, Sm-B/D, SMN and PRMT1 antibodies. ( d ) Reduced association between U1-snRNP with ALS-linked mutations in FUS/TLS. Extracts of isogenic lines expressing different GFP-tagged ALS-linked FUS/TLS mutations were immunoprecipiated with GFP antibodies and immunoblotted with antibodies against U1-A, U1-70K, Sm-B/D or CPSF-160. Decreased association of U1-70K and Sm-B/D with FUS/TLS was apparent in three of the four NLS mutations. Full size image Next, we determined how ALS-linked mutations in FUS/TLS affected association with U1-snRNP components, using isogenic cell lines expressing a single copy of LAP-tagged wild-type and ALS-linked FUS/TLS mutations R495X, R514G, R521G and P525L. While similar amounts of U1-A and CPSF-160 were co-immunoprecipitated with FUS/TLS for both wild-type and each mutant, the association of U1-70K and Sm-B/D (components of Sm core) was sharply reduced (by about fivefold) for the cytoplasmically mislocalized R495X and P525L, and the nuclear R521G mutant ( Fig. 5d ). U1-70K binding was selectively enhanced fivefold for R514G. However, the interaction with U1-A was not changed, suggesting that the increased binding was not with the whole U1-snRNP complex, which is essential for splice site recognition. Since U1-snRNP is also involved in preventing cryptic transcription termination [48] , it is possible the R514G mutant preferentially affects a different aspect of FUS/TLS function, such as polyadenylation. Mutations in FUS/TLS reduce activity on splicing regulation Since the altered association of FUS/TLS mutants with SMN and U1-snRNP could perturb splicing, we next tested whether the ALS-linked mutations in FUS/TLS affected alternative splicing. After inducing expression of GFP-tagged wild-type or mutant FUS/TLS in HeLa cells, endogenous FUS/TLS was reduced by transfection of an siRNA targeting a sequence in the 3′ untranslated region of the endogenous FUS/TLS gene, but missing from transgenes ( Fig. 6a ). Both wild-type and each of four ALS-causative mutations accumulated to levels comparable to the initial level of endogenous FUS/TLS ( Fig. 6b ). We then compared how many splicing events were altered by FUS/TLS depletion and if they were rescued by mutant FUS/TLS. For this, we exploited the RNA-mediated oligonucleotide annealing, selection and ligation with next-generation sequencing (RASL-seq) method, which permits quantitative profiling of several thousand selected alternative splicing events in a large number of samples [49] , [50] ( Fig. 6c ). Our probe library was assembled to assess 5,530 unique alternative splicing events, most of which were exon inclusion or skipping, with a minority for alternative 5′- or 3′- splice sites. Splicing profiling was performed on RNAs from three biological replicates in each group. Ratios of shorter to longer isoform counts were calculated and used to statistically compare the splicing changes between different groups ( Fig. 6d ). 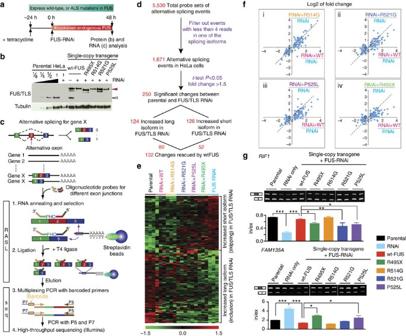Figure 6: ALS-linked mutations in FUS/TLS reduce its activity in alternative pre-mRNA splicing in HeLa cells. (a) Schematic timeline of endogenous FUS/TLS reduction and induction of GFP-tagged FUS/TLS, either wild type or with ALS mutations, in HeLa Flp-In cells. (b) Immunoblotting for FUS/TLS of cell extracts revealed replacement of endogenous FUS/TLS (white arrow) with comparable levels of various GFP-tagged FUS/TLS (red arrow). (c) Diagram of the RASL-seq methodology. (d) Flowchart illustrating the procedure of RASL-seq analysis and the number of alternative splicing events at each step. (e) Heatmap with hierarchical clustering of all the 132 wtFUS-rescued splicing events in groups of parental HeLa cells, cells with FUS/TLS knockdown (FUS RNAi), and replacement of endogenous FUS/TLS with GFP-tagged wild-type FUS/TLS (RNAi+WT), or R514G mutant FUS/TLS (RNAi+R514G), R521G mutant (RNAi+R521G), P525L (RNAi+P525L) or R495X (RNAi+R495X), with three biological replicates in each group. (f) Comparisons of rescue activities between various wild type and mutant FUS/TLS. The average fold changes of all the rescued splicing events were calculated by comparing the short to long isoform counts ratios in the group of RNAi+WT (or mutants) against the RNAi group. To evaluate how well FUS/TLS mutants rescued the splicing changes compared with the wild-type protein, the log2 of fold changes are presented in scatter plots. The dotted lines represent values with equal rescue between mutant and wild-type FUS/TLS. Note the decreased fold rescue (dots located between thexaxis and the dotted line) by three of the four NLS mutaions, consistent withf. (g) Validation of alternative splicing changes by RT–PCR. Quantification of splicing changes is from three biological replicates in each condition. *P<0.05, **P<0.01, ***P<0.001, one-way ANOVA using thepost hoctest; error bars represent s.e.m. Figure 6: ALS-linked mutations in FUS/TLS reduce its activity in alternative pre-mRNA splicing in HeLa cells. ( a ) Schematic timeline of endogenous FUS/TLS reduction and induction of GFP-tagged FUS/TLS, either wild type or with ALS mutations, in HeLa Flp-In cells. ( b ) Immunoblotting for FUS/TLS of cell extracts revealed replacement of endogenous FUS/TLS (white arrow) with comparable levels of various GFP-tagged FUS/TLS (red arrow). ( c ) Diagram of the RASL-seq methodology. ( d ) Flowchart illustrating the procedure of RASL-seq analysis and the number of alternative splicing events at each step. ( e ) Heatmap with hierarchical clustering of all the 132 wtFUS-rescued splicing events in groups of parental HeLa cells, cells with FUS/TLS knockdown (FUS RNAi), and replacement of endogenous FUS/TLS with GFP-tagged wild-type FUS/TLS (RNAi+WT), or R514G mutant FUS/TLS (RNAi+R514G), R521G mutant (RNAi+R521G), P525L (RNAi+P525L) or R495X (RNAi+R495X), with three biological replicates in each group. ( f ) Comparisons of rescue activities between various wild type and mutant FUS/TLS. The average fold changes of all the rescued splicing events were calculated by comparing the short to long isoform counts ratios in the group of RNAi+WT (or mutants) against the RNAi group. To evaluate how well FUS/TLS mutants rescued the splicing changes compared with the wild-type protein, the log2 of fold changes are presented in scatter plots. The dotted lines represent values with equal rescue between mutant and wild-type FUS/TLS. Note the decreased fold rescue (dots located between the x axis and the dotted line) by three of the four NLS mutaions, consistent with f . ( g ) Validation of alternative splicing changes by RT–PCR. Quantification of splicing changes is from three biological replicates in each condition. * P <0.05, ** P <0.01, *** P <0.001, one-way ANOVA using the post hoc test; error bars represent s.e.m. Full size image By comparing the groups of parental HeLa cells with the corresponding cells after reducing FUS/TLS, we identified a total of 250 events changed by decrease in FUS/TLS levels, including 124 increased long splicing isoforms and 126 enhanced short isoforms (defined by the t -test with P <0.05 and average fold change >1.5) ( Fig. 6d ; Supplementary Fig. 6b ). Inspection of heatmaps (produced with hierarchical clustering) revealed that expression of tagged wild-type FUS/TLS rescued the majority of splicing events that resulted from endogenous FUS/TLS reduction, yielding a pattern more similar to the parental cells ( Fig. 6e ). When comparing the groups with RNA interference (RNAi) of endogenous FUS/TLS in the presence of induced FUS/TLS transgenes to the groups with RNAi only, all ALS-linked mutations were found to rescue normal splicing less efficiently than wild-type FUS/TLS ( Fig. 6e ; Supplementary Table 2 ). The NLS truncation mutant R495X, which has the most severe cytosolic mislocalization ( Supplementary Fig. 6a ), failed almost completely to restore any splicing changes arising from suppression of endogenous FUS/TLS ( Fig. 6e ). Another severe NLS mutation (P525L) provided modestly better rescue of splicing changes, but was still far less efficient than wild-type FUS/TLS. Although both R514G and R521G mutants were primarily nuclear with no obvious cytoplasmic mislocalization ( Supplementary Fig. 6a ), they conferred different effects on splicing regulation. R514G activity was very similar to wild-type FUS/TLS, while R521G restored fewer splicing events, despite a higher accumulation level than R514G ( Fig. 6b,e ). Inspection of scatter plots of rescued fold changes also showed that rescue was worst for R495X and best for R514G, with the other two mutants in between ( Fig. 6f ). Multiple examples were validated by RT–PCR ( Fig. 6g ; Supplementary Fig. 6c ). Altogether, these results demonstrate that ALS-causative mutations in FUS/TLS acquire partial to nearly complete loss of normal function in regulating splicing. Interestingly, we also noticed that many of the splicing targets of FUS/TLS encode RBPs, or proteins involved in RNA metabolism ( Supplementary Table 3 ). Some splicing changes introduce premature stop codons and presumably induce nonsense-mediated decay of the mRNA (leading to reduced synthesis and function), while others modulate protein sequences in important domains ( Supplementary Table 3 ). These results indicate that there are probably extensive RNA processing defects in ALS patients with FUS/TLS mutations, both arising from direct effects of mutant FUS/TLS and indirect effects from altered activity of other RBPs whose levels or properties are changed by mutant FUS/TLS. A global RNA splicing signature in patient fibroblasts We next tested whether different FUS/TLS mutations conferred a common set of splicing changes when expressed from the normal human FUS/TLS locus. For this, we used RASL-seq to examine splicing alterations in three ALS patient fibroblasts with R521G, H517Q and M511Nfs*6 mutations in the FUS/TLS gene, and fibroblasts of three control individuals. Hierarchical clustering of short to long ratio for all events showed that the three FUS/TLS mutant lines clustered together and had a splicing profile distinct from control lines ( Supplementary Fig. 7 ). There were 57 splicing events found to have increased accumulation of a long isoform and 53 events have an enhanced short isoform (defined by the t -test P <0.05 and average fold change >1.5) ( Fig. 7a ; Supplementary Table 4 ). Inspection of heatmaps with hierarchical clustering of all these 110 splicing events identified splicing patterns common among three different FUS/TLS mutations ( Fig. 7b ). Several altered splicing events were validated using RT–PCR (along with four control individuals) ( Fig. 7c ), supporting a common RNA splicing signature in ALS patient cells with different FUS/TLS mutations. 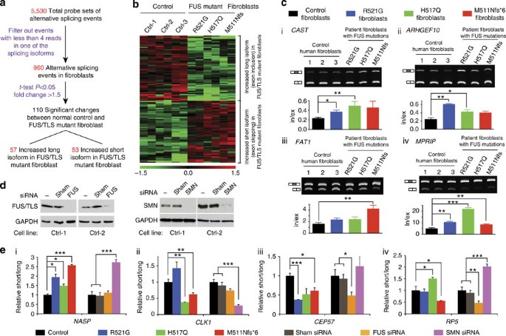Figure 7: RNA splicing profiling in human patient fibroblasts with FUS/TLS mutations. (a) Flowchart illustrating the procedure of RASL-seq analysis and the number of alternative splicing events at each step. (b) Heatmap with hierarchical clustering of 110 alternative splicing changes in the three patient fibroblasts with various FUS/TLS mutations compared with normal control fibroblasts, with duplicated samples in each cell line. (c) Validation of splicing changes by RT–PCR. Quantification for control is from five individual fibroblasts with duplicates each, two biological replicates for each FUS/TLS mutant. The group variance was analysed by one-way analysis of variance (ANOVA) followed by apost hoctest to determine the pairwise significant changes. *P<0.05, **P<0.01, ***P<0.001; error bars represent s.e.m. (d) Normal control fibroblasts were transfected with non-targeting siRNA or siRNA against FUS/TLS or SMN1 for 3 days. Immunoblotting of FUS/TLS and SMN showed the knockdown efficiency. GAPDH were blotted as internal control. (e) Comparison of splicing changes linked to FUS/TLS mutants with ones induced by FUS/TLS or SMN knockdown. Relative short to long isoform ratios are shown for 3 to 6 biological replicates in each condition. *P<0.05, **P<0.005, ***P<0.0005, one-way ANOVA using thepost hoctest; error bars represent s.e.m. Figure 7: RNA splicing profiling in human patient fibroblasts with FUS/TLS mutations. ( a ) Flowchart illustrating the procedure of RASL-seq analysis and the number of alternative splicing events at each step. ( b ) Heatmap with hierarchical clustering of 110 alternative splicing changes in the three patient fibroblasts with various FUS/TLS mutations compared with normal control fibroblasts, with duplicated samples in each cell line. ( c ) Validation of splicing changes by RT–PCR. Quantification for control is from five individual fibroblasts with duplicates each, two biological replicates for each FUS/TLS mutant. The group variance was analysed by one-way analysis of variance (ANOVA) followed by a post hoc test to determine the pairwise significant changes. * P <0.05, ** P <0.01, *** P <0.001; error bars represent s.e.m. ( d ) Normal control fibroblasts were transfected with non-targeting siRNA or siRNA against FUS/TLS or SMN1 for 3 days. Immunoblotting of FUS/TLS and SMN showed the knockdown efficiency. GAPDH were blotted as internal control. ( e ) Comparison of splicing changes linked to FUS/TLS mutants with ones induced by FUS/TLS or SMN knockdown. Relative short to long isoform ratios are shown for 3 to 6 biological replicates in each condition. * P <0.05, ** P <0.005, *** P <0.0005, one-way ANOVA using the post hoc test; error bars represent s.e.m. Full size image The mutant-dependent splicing alterations could arise from direct effects of compromising normal FUS/TLS splicing activity or indirectly through dysregulation of SMN function and/or through other RBPs, which are targets of FUS/TLS. To differentiate these effects, we next knocked down either FUS/TLS or SMN in control fibroblasts ( Fig. 7d ) and compared the splicing changes induced by acute loss of FUS/TLS or SMN proteins with splicing alterations in mutant FUS/TLS patient fibroblasts. We primarily focused on the M511Nfs*6 mutant as it is the most severe mutation. We observed 15 splicing changes induced by FUS/TLS knockdown and 8 changes induced by SMN knockdown in control fibroblasts that were also seen in M511Nfs*6 mutant cells ( Fig. 7e ; Supplementary Table 5 ). In most cases, one or both of the other mutants also had the same trend of alterations ( Fig. 7e ; Supplementary Table 5 ). We also identified another 12 splicing changes induced by SMN knockdown that had the opposite changes in FUS/TLS mutants. Three of the latter were regulated in opposite directions by FUS/TLS and SMN, and in this case some FUS/TLS mutants produced the same changes as reduction in FUS/TLS, while in other instances the changes mirrored loss of SMN ( Fig. 7e (iv)). The genetic background variation and combinatorial effects of different factors in patient fibroblasts, which have expressed the mutant FUS/TLS for a long time, make it difficult to systematically correlate with the effects from acute loss of FUS/TLS or SMN protein. Nevertheless, some splicing changes in mutant fibroblasts are consistent with the loss of FUS/TLS activity combined with dysregulation of SMN function. Combining quantitative mass spectrometry and affinity purification, we have identified FUS/TLS to be associated with SMN and U1-snRNP complexes. Remarkably, many NLS mutations in FUS/TLS yield an enhanced association with SMN, but a reduced binding to U1-snRNP, together affecting splicing regulation. Abnormally increased interaction of FUS/TLS with SMN might affect its normal nuclear and/or cytoplasmic dynamics and lead to Gem body reduction and dysregulation of snRNA levels, a potential common mechanism of SMN deficiency in SMA. The SMN complex acts as a chaperone to facilitate snRNP assembly in the cytoplasm [18] , [19] , [20] . Each of the snRNPs contains a unique snRNA and seven common Sm proteins, as well as a set of proteins specific to individual snRNAs. This function is mediated by binding of SMN to the Sm proteins through its Tudor domain, with the arginine-, glycine-rich (RG) domains on SmB, SmD and SmD3. In the nucleus, SMN-containing Gem bodies partially and dynamically associate with Cajal bodies mediated by the interaction between SMN’s Tudor domain and the RG dipeptide motif in Coilin [51] , which might be essential for snRNP maturation and cycling. Despite the complexity of SMN functions in vivo , snRNP metabolism is impaired with SMN deficiency in SMA, and the various snRNA levels are also altered to different degrees in different tissues or conditions [22] , [24] , [25] , [26] , [27] . Our evidence has shown FUS/TLS to directly bind SMN, mediated by the three RGG motifs in FUS/TLS and the single Tudor domain in SMN, the key motif for interaction with many partners. It is possible that the increased binding with mutant FUS/TLS interferes with the normal dynamics of SMN complex assembly and/or trafficking/cycling, therefore leading to dysregulation of SMN function. Furthermore, this disruptive feature might be facilitated by the aggregation-promoting prion-like feature of FUS/TLS [52] . The association of FUS/TLS with U1-snRNP and two other splicing factors, SRSF1 and SRSF3, is consistent with the role of FUS/TLS in RNA splicing. Reduction of association between FUS/TLS mutants with U1-snRNP suggests a loss of activity in splicing regulation by FUS/TLS. The two mutants (P525L and R495X) that were mislocalized in the cytoplasm have more severe splicing defects accompanied with their reduced interaction with U1-snRNP. Comparing two mainly nuclear mutants (R521G and R514G) with reduced and enhanced binding to U1-snRNP, respectively, the reduced interaction of R521G correlated with its inability to complement the loss of endogenous FUS/TLS. These findings indicate that some ALS-linked mutations in FUS/TLS lead to defects in its nuclear function, independent of cytosolic redistribution, and strongly suggest that the interaction of FUS/TLS with U1-snRNP is directly involved in FUS/TLS splicing activity. It also should be noted that CPSF-160 and PABPC1 are two proteins in the FUS/TLS interactome that are involved in 3′-end RNA processing. We further showed that FUS/TLS, U1-snRNP and CPSF-160 may indeed form a large complex (~1.8 MDa). This is particularly intriguing, as the recent work uncovered that U1-snRNP may serve as a governing machinery for blocking premature polyadenylation [48] , suggesting FUS/TLS might play an important role in regulating polyadenylation selection. In addition, three ALS-linked genes, EWSR1 , TAF-15 and TDP-43 , are components of the FUS/TLS interactome. It has been previously demonstrated that a small proportion of TDP-43 interacts with FUS/TLS [37] . Interestingly, EWSR1 and TAF-15 co-aggregate with FUS/TLS in FTD patients with FUS pathology, but apparently not in ALS patients with FUS mutations [53] . Determining the significance of EWSR1 and TAF-15 association will require further investigation. Finally, we have identified a common RNA splicing signature profile in ALS patient fibroblasts carrying three different mutations in FUS/TLS. Although we previously reported splicing changes caused by FUS/TLS depletion in mouse brain [11] , the differences in species and cell types make comparison problematic. We therefore reduced either FUS/TLS or SMN in control fibroblasts and compared the corresponding changes with those in mutant FUS/TLS fibroblasts. Although there was no expectation that acute loss of function would match that from chronic reduction, we still observed several splicing alterations in the mutant fibroblasts that showed the same trends as the changes produced by FUS/TLS or SMN knockdown. Interestingly, while FUS/TLS mutant-linked splicing changes always showed the same direction of changes as in FUS/TLS knockdown conditions, half of the overlaps with SMN knockdown occurred in opposite directions, suggesting the effect on SMN function might be more complicated than pure loss of activity. In addition, the disease-related splicing changes may arise from synergetic effects of direct effects (from reduced splicing activity of mutant FUS/TLS and/or its altered recognition of specific pre-mRNA substrates) and indirect effects (altered U-snRNP metabolism and altered expression levels of other RBPs, which are targets of FUS/TLS). Taken together, our work has detailed that FUS/TLS interacts with SMN and U1-snRNP ( Fig. 8 ). ALS-causative mutations in FUS/TLS affect SMN function as indicated by reduced Gem bodies and altered snRNP metabolism, potentially through abnormal interaction of SMN with its normal partners and compromised localization, dynamics or function of SMN complexes, thereby representing a potential ‘gain of FUS/TLS toxicity’. The same mutations also lead to a reduced activity of FUS/TLS in regulated alternative splicing accompanied by a reduced interaction with U1-snRNP, that is, a ‘loss-of-function’ effect. Both of the ‘gain’ and ‘loss’ properties are independent of obvious cytosolic mislocalization, although the defects tend to be worse in mutants with more cytosolic distribution. Abnormal copy numbers (one or three copies) of the SMN1 gene have been associated with significantly increased risk of sporadic ALS [54] . Mutations in FUS/TLS (especially ones disrupting the NLS) have also been linked recently to juvenile-onset ALS [55] , [56] , a disease closer in form to SMA3 (juvenile SMA, the mildest form of SMA). The collective evidence supports a convergent pathological pathway in which defects in RNA metabolism may be central mechanistic components to ALS and SMA, the most prominent motor neuron diseases in adults and children, respectively. 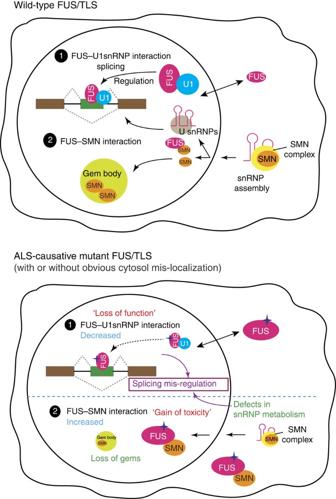Figure 8: Diagram for molecular mechanisms underlying gain and loss of RNA-processing functions by ALS-causative mutations in FUS/TLS. ALS-causative mutations in FUS/TLS enhance the interaction with SMN, potentially sequestering SMN from its normal localization and function, thereby reducing Gem bodies, affecting snRNP assembly, and therefore affecting downstream RNA processing, a ‘gain of toxicity’. The same mutations also decrease FUS/TLS interaction with U1-snRNP, which leads to reduced activity of FUS/TLS in mediating alternative splicing, a ‘loss-of-function’ effect similar to loss of wild-type FUS/TLS. Figure 8: Diagram for molecular mechanisms underlying gain and loss of RNA-processing functions by ALS-causative mutations in FUS/TLS. ALS-causative mutations in FUS/TLS enhance the interaction with SMN, potentially sequestering SMN from its normal localization and function, thereby reducing Gem bodies, affecting snRNP assembly, and therefore affecting downstream RNA processing, a ‘gain of toxicity’. The same mutations also decrease FUS/TLS interaction with U1-snRNP, which leads to reduced activity of FUS/TLS in mediating alternative splicing, a ‘loss-of-function’ effect similar to loss of wild-type FUS/TLS. Full size image Plasmids FUS/TLS cDNA was subcloned into pcDNA-Flag via BamHI and XhoI sites. The RGG1 (aa 213–261), RGG2 (aa 377–407), RGG3 (aa 473–505), RRM (aa 285–370) or NLS (aa 514–525) domains were deleted, and ALS-linked point mutations were introduced by QuickChange mutagenesis. SMN was subcloned into pcDNA-HA via BamHI and XhoI sites and the Tudor domain (aa 95–143) deleted by QuickChange mutagenesis. FUS/TLS was subcloned into pGEX6p-1 using BamHI and SalI sites to generate an N-terminal GST-fusion tag. The Flp-In LAP-tag constructs based on pcDNA5/FRT/TO were as described [37] . In brief, N-terminal HA-peptide (YPYDVPDYA)-tagged FUS/TLS was amplified by PCR and inserted into pcDNA5/TO/FRT/LAP using XhoI and NotI sites. ALS-linked mutations were generated by QuickChange mutagenesis (Stratagene) and confirmed by sequencing the entire open-reading frame. Cell culture and transfection HeLa, N2a and NSC34 cells were grown in Dulbecco’s modified Eagle’s medium (DMEM) supplemented with 10% (v/v) fetal bovine serum (FBS), 100 U ml −1 penicillin and 100 μg ml −1 streptomycin. Primary human fibroblasts ( Supplementary Table 6 ) were grown in DMEM supplemented with 20% FBS, 0.1 mM nonessential amino acids (Invitrogen), 2 mM L -glutamine (Invitrogen) and penicillin/streptomycin. For differentiation of N2a cells into neuronal-like cells, N2a were cultured in DMEM with 2% FBS and 20 μM retinoic acid for 4 days. X-tremeGENE 9 (Roche) was used to transfect plasmids; Lipofectamine RNAiMAX (Invitrogen) was used to transfect siRNAs. For knockdown experiments, siRNAs were transfected 72 h prior to sample collection. The siRNA for FUS/TLS was designed to target the 3′ untranslated region (5′- GACUAUGUAAUUGUAACUAUA -3′). The siRNA for SMN1 was designed to target 5′- GAAGAAUACUGCAGCUUCCUUAC -3′. ON-TARGETplus Non-Targeting siRNA (Dharmacon) was used as a negative control. The isogenic HeLa stable cell lines expressing FUS/TLS transgenes were generated as described before [37] . Transgene expression was induced with 4 μg ml −1 tetracycline for 72 h. For replacement experiments, isogenic HeLa cell lines were induced with tetracycline overnight prior to siRNA transfection. Affinity purification and quantitative mass spectrometry The procedure for TAP-SILAC was performed as before [37] . Cells were grown in SILAC DMEM (Thermo Scientific) supplemented with 10% dialysed FBS and penicillin/streptomycin with 0.4 mM of L -arginine and 0.8 mM of L -lysine. Normal (‘light’) L -arginine (69.2 μg ml −1 ) and L -lysine (116.6 μg ml −1 ) were added to the ‘light’ growth medium, and ‘heavy’ L-Arg- 13 C 6 , 15 N 4 .HCl (87.8 μg ml −1 ) and L-Lys- 13 C 6 , 15 N 2 .HCl (152 μg ml −1 ) were added for the ‘heavy’ growth medium. For the forward and reverse SILAC, stable Flp-In cell lines expressing either wild-type or ALS-linked mutations in FUS/TLS were cultured with either light or heavy medium as indicated. Immunofluorescence, immunoblotting and antibodies For HeLa and N2a cells, cells were fixed with 4% (v/v) paraformaldehyde in PBS for 20 min. Cells were permeabilized in 0.2% (v/v) Triton X-100 for 5 min, blocked in 1% bovine serum albumin and 2% donkey serum for 30 min., incubated with primary antibodies for 1 h, washed with PBS and finally incubated with FITC- or Cy3- conjugated secondary antibodies (Jackson ImmunoResearch). Nuclei were counterstained with 4,6-diamidino-2-phenylindole. Cells were imaged with a DeltaVision-modified inverted microscope (IX70; Olympus). For human fibroblasts, cells were fixed with methanol/acetone (1:1) for 15 min, permeabilized in 0.1% (v/v) Triton X-100 for 15 min and incubated with primary antibodies overnight at 4 °C. The quantification of Gems was represented as the average Gem numbers per cell in each cell line with three biological replicates. One-way analysis of variance was used to assess the variation among individual cell lines, showing the variation was not statistically significant within control cell lines, while it was comparing controls versus mutants. For immunoblotting, goat anti-mouse or anti-rabbit IgG HRP conjugate (GE healthcare) was used along with chemiluminescent detection reagents (Thermo Scientific). The primary antibodies included GAPDH (Cell Signaling, #2118, 1:5,000), Flag tag (Sigma, F3165, 1:500), HA tag (Novus, NB600-363, 1:1,000), FUS/TLS (Bethyl, A300-302A, 1:5,000; Santa Cruz, sc-47711, 1:500), SMN (BD, #610646, 1:5,000), U1-70K (Millipore, 1:2,000), U1-A (Abnova, H00006626-D01P, 1:2,000), U1-C (Sigma, SAB4200188, 1:1,000), Sm-B/D (Thermo, MS-450-P0, 1:250), CPSF-160 (Bethyl, A301-580A, 1:5,000), PABPC1 (Santa Cruz, sc-32318, 1:100), GEMIN5 (Bethyl, A301-325A, 1:5,000), HSP90 (Stressgen, ADI-SPA-846, 1:3,000), Histone H3 (Sigma, H0164, 1:5,000). The listed concentration was used for immunoblotting, and five- to ten-fold less diluted for immunofluorescence. Tissue preparation and the procedure for immunohistochemistry was described previously [57] . In brief, anesthetized mice were transcardialy perfused with PBS, followed by 4% paraformaldehyde (PFA) in phosphate buffer for fixation. Spinal cords were post-fixed in 4% paraformaldehyde for 2 h, cryoprotected in 30% sucrose for over 24 h and embedded in Tissue-Tek. Fixed spinal cords were sectioned at 30 μm thickness for staining. Antigen retrieval treatment was used for SMN staining, in which tissue sections were immersed in 10 mM sodium citrate (pH 6.0) at 95 °C for 15–20 min. Sections were cooled down to room temperature and rinsed extensively with PBS before proceeding to immunofluorescence staining. Immunoprecipitation Dynabeads Protein G were washed twice with citrate-phosphate buffer (25 mM citric acid, 50 mM Na 2 HPO 4 , pH 5.0), and incubated with FUS/TLS antibody for 1 h at room temperature. The beads were washed twice in 500 μl citrate-phosphate buffer, and once in immunoprecipitation (IP) lysis buffer (0.3% (v/v) NP-40, 200 mM NaCl, 50 mM Tris, pH 7.4, 1 mM dithiothreitol, 0.1 mM EDTA, 0.1 mM EGTA, with freshly added 1 mM sodium vanadate, 50 mM sodium fluoride and a protease-inhibitor cocktail). Anti-FLAG M2 affinity gel (Sigma, A2220) was used for FLAG IP; GFP-binding for GFP IP [35] , [58] . Individual 15-cm plates of HeLa cells were lysed in 1 ml of IP lysis buffer, and the DNA sheared by a sequential passage through a syringe with 20G, 22G and 26G needles, three times each. The lysates were clarified by centrifugation at 13,000g for 20 min at 4 °C. The supernatants were passed through a 0.45-μm filter (Costar). We then added 20 μl beads (1:1 suspension) to the cleared lysates and incubated for 4 h at 4 °C. After washing five times in lysis buffer, the beads were resuspended in SDS-containing gel sample buffer and electrophoresed on an SDS–polyacrylamide gel electrophoresis (PAGE) gel. For RNase treatment, a nuclease cocktail (1 U ml −1 RNase cocktail (Ambion), 500 U ml −1 Benzonase (Novagen) and 2 mM MgCl 2 ) was added and incubated on ice for 30 min. For cell fractionation before IP, cells were gently lysed (in 20 mM Tris pH 7.4, 10 mM NaCl, 3 mM MgCl 2 , 0.3% (v/v) NP-40, 1 mM dithiothreitol, 0.1 mM EDTA, 0.1 mM EGTA, with freshly added 1 mM sodium vanadate, 50 mM sodium fluoride and protease-inhibitor cocktail). Nuclei were pelleted at 2,300 g for 5 min at 4 °C, and transferred to a new tube. The nuclei were washed once with the same buffer, re-pelleted and resuspended in IP lysis buffer. Both nuclear and cytosol fractions were clarified at 15,000 r.p.m. for 20 min. We adjusted the cytosolic fraction to 200 mM NaCl and proceeded for immunoprecipitation. Recombinant protein purification and GST pull-down assay GST-tagged recombinant proteins were purified using glutathione sepharose following the manufacture’s protocol (GE healthcare). Coupled in vitro transcription and translation reactions were used to generate SMN and delta-Tudor SMN proteins with 35 S-methione and cysteine (Promega). Purified GST and GST-FUS (500 ng) were incubated with SMN and delta-Tudor SMN together with 20 μl of glutathione sepharose at 4 °C for 1 h. The beads were subsequently washed three times with wash buffer (50 mM HEPES, pH 7.5, 150 mM KCl, 1 mM MgCl2, 0.1% NP-40 and 10% glycerol). The associated proteins were eluted with 15 mM glutathione and analysed by autoradiography. 6 × His-tag recombinant proteins were expressed in bacteria and purified with Ni-NTA (Qiagen) according the manufacturer’s manual. The in vitro GST pull-down assay using GST, GST-FUS and GST-TDP-43 with equal amount of recombinant SMN proteins performed as described above. The associated proteins were eluted with 15 mM glutathione and analysed with immunoblots. Gel filtration chromatography High-speed supernatant from HeLa cells were prepared as described for TAP-SILAC. Fifteen mg of HSS is loaded onto Superose 6 column (GE Healthcare) equilibrated in 20 mM Tri-HCl, pH 7.4, 50 mM KCl, 1 mM MgCl 2 . Fractions of 1 ml were collected immediately after the void volume and analysed by immunoblotting as indicated in the figure legend. The calibration of the size-exclusion column was performed with the following molecular weight markers: blue dextran (2 MDa), thyroglobulin (670 kDa), ferritin (440 kDa), aldolase (158 kDa) and ovalbumin (44 kDa). Peak fractions of the molecular weight markers are indicated in Fig. 5c . RNA isolation, qRT–PCR and RT–PCR To isolate total RNA from cells or tissues, Trizol (Invitrogen) and treatment with RQ1 DNase I (Promega) was used. For first-strand cDNA synthesis, random hexamers were used with the High-capacity cDNA reverse transcription kit (Applied Biosystems). All qRT–PCR reactions for snRNAs were performed with three biological replicates for each group and two technical replicates using the iQ SYBR green supermix (Bio-Rad) on the iQ5 multicolour real-time PCR detection system (Bio-Rad). The data were analysed using the iQ5 optical system software (Bio-Rad; version 2.1). Expression values were normalized to two control genes: 5S rRNA and 5.8S rRNA . Expression values were expressed as a percentage of the average expression of control samples. Regular RT–PCR (25–30 cycles) was used to validate alternative splicing changes. Isoform products were separated on 10% polyacrylamide gels and stained with SYBR gold (Invitrogen) and quantified with Image Lab (Bio-Rad). Intensity ratios of long and short isoforms were averaged from three biological replicates per group. PCR primer sequences are shown in Supplementary Table 7 . For experiments using patient fibroblasts, one-way analysis of variance was used to assess variations among control and mutant cell lines. Genes with significant variations ( P <0.05) were further analysed by a post hoc test to determine the pairwise significant changes. RASL-seq RASL-seq analysis of splicing switches was carried out as detailed [49] , [50] . A pool of oligonucleotides was designed to detect 5,530 alternative splicing events in human. One hundred fmol of RASL-seq oligos were annealed to 1 μg of total RNA isolated from HeLa or human fibroblast cells. After ligation, 5 μl eluted ligated oligos was used for 16~20 cycles of PCR amplification, and the bar-coded PCR products were sequenced on HiSeq2000 with 24–30 samples in one lane. Sequencing data were decoded allowing no mismatch with each barcode, and target sequences were mapped with RASL-seq oligo pool sequences with Bowtie [59] allowing for one mismatch. An average of 5 million reads from each sample was mapped, with events with <4 counts in one of the isoforms removed. Ratios of the counts of shorter to longer isoforms were calculated. The significantly changed events were identified by the t -test and average fold change. Heatmaps were generated by hierarchical clustering and TreeView [60] . How to cite this article : Sun, S. et al . ALS-causative mutations in FUS/TLS confer gain and loss of function by altered association with SMN and U1-snRNP. Nat. Commun. 6:6171 doi: 10.1038/ncomms7171 (2015). Accession codes: The raw data of RASL-seq have been deposited in Gene Expression Omnibus (GEO) under the accession code GSE64078 .